Anti-infective therapy using species-specific activators ofStaphylococcus aureusClpP The emergence of methicillin-resistant Staphylococcus aureus isolates highlights the urgent need to develop more antibiotics. ClpP is a highly conserved protease regulated by ATPases in bacteria and in mitochondria. Aberrant activation of  bacterial ClpP is an alternative method of discovering antibiotics, while it remains difficult to develop selective Staphylococcus aureus ClpP activators that can avoid disturbing Homo sapiens ClpP functions. Here, we use a structure-based design to identify ( R )- and ( S )-ZG197 as highly selective Staphylococcus aureus ClpP activators. The key structural elements in Homo sapiens ClpP, particularly W146 and its joint action with the C-terminal motif, significantly contribute to the discrimination of the activators. Our selective activators display wide antibiotic properties towards an array of multidrug-resistant staphylococcal strains in vitro, and demonstrate promising antibiotic efficacy in zebrafish and murine skin infection models. Our findings indicate that the species-specific activators of Staphylococcus aureus ClpP are exciting therapeutic agents to treat staphylococcal infections. S taphylococcus aureus ( S. aureus ) colonizes the human skin and nares and frequently causes invasive and life-threatening diseases [1] . Methicillin-resistant S. aureus (MRSA) is responsible for many hospital-acquired infections, which include surgical site infections, bacteremia, and sepsis [2] . MRSA has acquired multidrug resistance against many antibiotics, including β-lactam, cephalosporin, fluoroquinolone, aminoglycoside, tetracycline, macrolide, and trimethoprim-sulfamethoxazole [3] . Due to this resistance, antibiotic prophylaxis of MRSA infections frequently incites nosocomial diseases such as Clostridium difficile infection [4] . Given the dwindling supply of potent antibiotics, it is increasingly important to develop new methods of treating multidrug-resistant MRSA infections [5] . To this end, developing antistaphylococcal agents, particularly those with a different mode of action, is urgently needed to provide future treatments for MRSA infections [6] , [7] , [8] , [9] , [10] , [11] . Caseinolytic protease P (ClpP) is a highly conserved protease regulated by ATPases in bacteria and in human mitochondria, and plays an important role in protein quality control by regulating and degrading the misfolded or damaged proteins [12] , [13] . In bacteria, ClpP is responsible for modulating the expression of virulence factors, antibiotic resistance, and the formation of biofilms and persisters [14] , [15] , [16] , [17] . Likewise, Homo sapiens ClpP ( Hs ClpP), which is found in the mitochondria, is a key protease regulating mitochondrial proteins homeostasis. These proteins are mainly involved in respiratory chain complexes [18] . The dysregulated expression or tissue distribution of Hs ClpP is strongly associated with diseases, such as cancer and neurological disorders [19] , [20] . The dysfunction of ClpP by small molecule activators has recently been demonstrated to be a possible method of discovering antibacterial and anticancer drugs [21] . Remarkably, acyldepsipeptides (ADEPs) has been identified as a promising class of antibiotics, which reveal that bacterial ClpP is a possible antibiotic drug target [22] , [23] . These naturally occurring activators allosterically switch S. aureus ClpP ( Sa ClpP) to a gain-of-function state to degrade multiple essential proteins, such as the filamentous temperature-sensitive Z ( Sa FtsZ), which inhibits cell division and eventually leads to bacterial cells death [24] , [25] . In addition, ADEP 4 suppresses the growth of persisters and eradicates a chronic biofilm infection when combined with marketed antibiotics [23] , indicating that the therapeutic application of ADEPs can be used in combination therapy. However, the chemical instability issues of ADEP analogs could significantly restrict the applications of antibiotic drug discovery [26] . The discovery of ADEPs as bacterial ClpP activators has inspired studies on Hs ClpP. The aberrant activation of Hs ClpP protease activity significantly degrades multiple proteins in the respiratory chain complex, which exerts antitumor effects [27] . Of note, ADEP-28, an analog of ADEP 4, was shown to activate Hs ClpP and induce cytotoxic effects by activating intrinsic, caspase-dependent apoptosis [28] . Additionally, imipridone ONC201 and ONC212 activate the Hs ClpP protease and facilitate ClpP-mediated proteolysis, resulting in cancer cell lethality [27] , [29] . ONC212 also functions as an antibiotic, which activates ClpPs from Escherichia coli , Bacillus subtilis , and S. aureus in biochemical and genetic assays and eventually suppressed bacterial cell proliferation [30] . Recently, we found that ONC212 and ADEP 4 dysregulated Xoo ClpP to degrade Xoo FtsZ, which suggests a promising strategy of treating leaf blight diseases [31] . Other activators, such as bengamide analogs and activators of self-compartmentalizing proteases (ACPs), also exhibit certain activities on ClpP [32] , [33] , [34] . However, to date, there is no species-specific activator for the Sa ClpP protease. In this study, we report on two highly selective Sa ClpP activators, ( R )- and ( S )-ZG197, which selectively activates Sa ClpP rather than Hs ClpP. Additionally, ( R )-ZG197 exhibits a broad range of antibiotic properties towards an array of MRSA strains and shows promising antibiotic efficacy in vivo. Identification of ZG180 as a Sa ClpP activator Since ADEP 4 and ONC212 are global activators for ClpP proteases (Supplementary Fig. 1a ), our goal is to develop small molecule activators that selectively enhance the Sa ClpP protease activity over Hs ClpP (Fig. 1a ). Given the established structure-activity relationships of ADEP 4 and ONC212 as ClpP activators [29] , [35] , [36] , [37] , [38] , we search for distinct chemical scaffolds as selective activators for Sa ClpP. To this end, we conducted a high-throughput screening (HTS) on a compound library containing 3,896 candidates. ICG-001 was confirmed to promote hydrolysis of the fluorescein isothiocyanate-labelled casein (FITC-casein) in the presence of Sa ClpP (Supplementary Fig. 1b and 1c ). ICG-001 was initially characterized as a Wnt signaling pathway inhibitor, while it was recently screened as an activator for Hs ClpP [39] , [40] . Considering distinct scaffold of ICG-001 and the practicable synthesis of derivatives, we chose ICG-001 as a starting point for follow-up synthetic optimization [41] . Incorporation with the isoleucine fragment and 4,4,4-trifluorobutyl motif into the core scaffold of ICG-001 provided a potent ClpP activator ZG180 (Fig. 1b ). ZG180 is more potent than ICG-001 in activating Sa ClpP for α-casein hydrolysis, as evidenced by a 3-fold decrease in EC 50 (Fig. 1c and Supplementary Fig. 1d ). However, ZG180 also promotes Hs ClpP for α-casein hydrolysis (Fig. 1c and Supplementary Fig. 1e ), which indicates that ZG180 is also a global activator for both bacterial and mitochondrial ClpP proteins. Fig. 1: Identification of ZG180 as potent ClpP activator. a The goal of this work is to develop selective Sa ClpP activators. b The synthetic lead compound ZG180 as ClpP activator. c Quantitation of α-casein hydrolysis by Sa ClpP and Hs ClpP in the presence of ICG-001 and ZG180, respectively ( n = 3 biologically independent experiments). Data are presented as mean ± SD (error bars). X-ray crystal structure of ZG180/ Sa ClpP ( d ) and ZG180/ Hs ClpP ( e ) complexes. Side and top views of the structural complexes are displayed. Sa ClpP is shown in gray cartoon tube, Hs ClpP is shown in wheat cartoon tube, and ZG180 is shown in cyan sphere. f , g The electron density maps and close view of ZG180 binding in the hydrophobic pockets of Sa ClpP ( f ) and Hs ClpP ( g ). The fo-fc omit map is contoured at 3.0 Å and colored in green, while the 2fo-fc map is contoured at 1.0 Å and colored in magenta. ZG180 is shown in cyan stick. Hydrogen bonds are indicated with dark dashed lines, and the distance in Å is labeled. Source data are provided as a Source Data file. 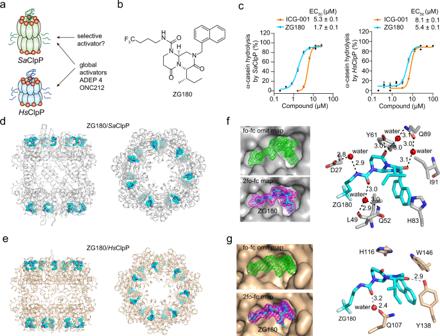Fig. 1: Identification of ZG180 as potent ClpP activator. aThe goal of this work is to develop selectiveSaClpP activators.bThe synthetic lead compound ZG180 as ClpP activator.cQuantitation of α-casein hydrolysis bySaClpP andHsClpP in the presence of ICG-001 and ZG180, respectively (n= 3 biologically independent experiments). Data are presented as mean ± SD (error bars). X-ray crystal structure of ZG180/SaClpP (d) and ZG180/HsClpP (e) complexes. Side and top views of the structural complexes are displayed.SaClpP is shown in gray cartoon tube,HsClpP is shown in wheat cartoon tube, and ZG180 is shown in cyan sphere.f,gThe electron density maps and close view of ZG180 binding in the hydrophobic pockets ofSaClpP (f) andHsClpP (g). The fo-fc omit map is contoured at 3.0 Å and colored in green, while the 2fo-fc map is contoured at 1.0 Å and colored in magenta. ZG180 is shown in cyan stick. Hydrogen bonds are indicated with dark dashed lines, and the distance in Å is labeled. Source data are provided as a Source Data file. Full size image To investigate the molecular mechanism of our activator-promoted proteolysis of ClpP proteases, we resolved the crystal structure of ZG180 bound to Sa ClpP (7WID in PDB) and Hs ClpP (7WH5 in PDB) to a resolution of 1.90 Å and 2.13 Å, respectively (Supplementary Table 1 ). Either ZG180/ Sa ClpP or ZG180/ Hs ClpP structure is a single tetradecamer composed of two stacked heptameric rings (Fig. 1d, e ). Like the previously characterized ClpP activators, the binding of fourteen ZG180 molecules induces an open-gated state in the tetradecameric ClpP cylinders with an enlarged axis entrance pore [42] , [43] , [44] , [45] . The apparent electron densities in the 2fo-fc and fo-fc omit maps unambiguously demonstrate ZG180 binding on the apical surface of Sa ClpP and Hs ClpP (Fig. 1f, g ). The naphthyl motif and trifluorobutyl chain in ZG180 form hydrophobic stacking in the binding pockets of Sa ClpP, which contributes to the enhanced interactions. A network of hydrogen bonds between ZG180 and the side chains of D27, L49, Q52, Y61, and Q89 collectively increase the binding affinity to Sa ClpP (Fig. 1f ). A similar binding manner is observed in the ZG180/ Hs ClpP structure (Fig. 1g ). These structural features are similar to the previously reported structural complexes of both Sa ClpP and Hs ClpP bound with small molecule activators, such as ADEP 4/ Sa ClpP, ADEP-28/ Hs ClpP, and ONC201/ Hs ClpP [27] , [28] , [35] , in which all the activator molecules are similarly positioned in the hydrophobic pockets and prevent ATPase binding to ClpP. Development of ( R )- and ( S )-ZG197 as selective Sa ClpP activators by structure-based design To design a specific activator for Sa ClpP over Hs ClpP, we analyzed the amino acid sequences that can affect the binding mode of ZG180 in two ClpP proteins. While Sa ClpP and Hs ClpP share a high similarity in the primary sequences (Supplementary Fig. 2a ), there is a large indole motif of W146 in Hs ClpP but a much smaller isopropyl side chain of I91 in Sa ClpP in the conserved position. Indeed, structural superimposition of the ZG180/ Sa ClpP and ZG180/ Hs ClpP complexes also reveals that the α-carbon of the naphthyl motif in ZG180 is likely to be a discriminant site for introducing steric clash against the bulky side chain of W146 in Hs ClpP (Fig. 2a ). To this end, we incorporated a methyl group on ZG180 to obtain two naphthalen-1-ylmethyl analogs ( R )- and ( S )-ZG197 (Fig. 2b ). Similar to ZG180, both ( R )-ZG197 and ( S )-ZG197 activate Sa ClpP to degrade α-casein and Sa FtsZ in vitro (Fig. 2c , Supplementary Fig. 2b, c ). Unlike the nonselective ZG180 activator, ( R )-ZG197 activates Sa ClpP with an EC 50 value of 1.5 μM that is a 20-fold higher activity than that activates Hs ClpP, while ( S )-ZG197 fails to activate Hs ClpP even at 100 μM (Fig. 2c and Supplementary Fig. 2d ). Moreover, both ( R )-ZG197 and ( S )-ZG197 promote the degradation of cellular Sa FtsZ protein in cell lysates of S. aureus 8325-4 clpP knockout (Δ clpP ) strain with the supplement of the recombinant Sa ClpP protein, but no Sa FtsZ degradation occurred in the presence of the recombinant Hs ClpP protein. In contrast, the global activator ONC212 activates both Sa ClpP and Hs ClpP to degrade the cellular Sa FtsZ protein (Fig. 2d ). In conclusion, by using structure-based design, we successfully developed the species-specific Sa ClpP activators ( R )- and ( S )-ZG197 that minimally disturb the activity of mitochondrial ClpP in vitro. Fig. 2: Design and development of selective Sa ClpP activators. a Structural superimposition of ZG180/ Sa ClpP and ZG180/ Hs ClpP complexes to reveal the strategy for designing selective activators for Sa ClpP over Hs ClpP. Sa ClpP and Hs ClpP are shown in gray and wheat cartoon tubes, respectively. ZG180 is colored in cyan in the ZG180/ Sa ClpP structure, while it is colored in yellow in the ZG180/ Hs ClpP structure. I91 in Sa ClpP and W146 in Hs ClpP are shown as a stick. b Structures of Sa ClpP activators ( R )- and ( S )-ZG197 developed by the structure-based design outlined in ( a ). The chiral methyl group is indicated in red. c Quantitation of α-casein hydrolysis by Sa ClpP and Hs ClpP in the presence of ( R )- and ( S )-ZG197, respectively ( n = 3 biologically independent experiments). Data are presented as mean ± SD (error bars). d Effect of activators on degradation of the cellular Sa FtsZ protein with the supplement of bovine serum albumin (BSA), the recombinant Sa ClpP, and Hs ClpP, respectively, in cell lysates of the clpP deletion (Δ clpP ) mutant. The abundance of cellular Sa FtsZ is quantitated with a Western blot assay. Quantitation on the band intensity of Sa FtsZ is normalized against the loading control of Sa GAPDH, and the ratio in the DMSO group is considered as 1.0. Source data are provided as a Source Data file. Full size image Characterization on the interactions between our activators and Sa ClpP To explain why our activators selectively activate Sa ClpP rather than Hs ClpP in vitro, we measured the direct interactions between ( R )- or ( S )-ZG197 compounds and the two ClpP proteases. During the differential scanning fluorimetry (DSF) analysis, ( R )-ZG197 significantly enhances the thermal stability of Sa ClpP in a dose-dependent manner while having a weak effect on Hs ClpP (Fig. 3a ). This indicates that ( R )-ZG197 exhibited a stronger binding affinity for Sa ClpP than Hs ClpP. Similarly, ( S )-ZG197 increases the melting temperature (T m ) of Sa ClpP but barely changes the T m of Hs ClpP (Fig. 3b ). We then conducted an isothermal titration calorimetry (ITC) assay to determine the stoichiometries of the binding capacity. The dissociation constant ( K d ) for ( R )- and ( S )-ZG197 binding to Sa ClpP is quantitatively estimated to be 2.5 ± 0.2 μM and 5.0 ± 0.3 μM, respectively (Fig. 3c ). We also analyzed our activators’ binding to Sa ClpP and Hs ClpP in biolayer interferometry (BLI). Likewise, ( R )- and ( S )-ZG197 display a K d of 58 ± 4.8 nM and 470 ± 60 nM for binding to Sa ClpP, respectively (Supplementary Fig. 3a ). However, neither ( R )-ZG197 nor ( S )-ZG197 exhibits detectable binding affinity to Hs ClpP in BLI analysis (Supplementary Fig. 3b ). This indicates that our activators selectively bind to Sa ClpP rather than Hs ClpP in vitro. Fig. 3: Investigation of the interaction between species-selective activators and Sa ClpP. Effect of ( R )- ( a ) and ( S )-ZG197 ( b ) on the thermal stability of Sa ClpP and Hs ClpP in DSF assay, respectively. T m , melting temperature. c Determination of ( R )- and ( S )-ZG197 binding to Sa ClpP by ITC titration. The dissociation constant ( K d ) and stoichiometry factor (N) are indicated. Effect of activators on the thermal stability of the cellular Sa ClpP ( d ) and Hs ClpP ( e ), respectively. The S. aureus 8325-4 was cultured in the presence of 10 μM compound for 2 h before running CETSA ( d ), while cell lysates of HEK 293 T/17 were assayed in CETSA ( e ). The proteins in unheated samples are used as inputs and considered as 100%. Data ( a , b , d , and e ) are obtained from three biologically independent experiments and presented as mean ± SD (error bars). Source data are provided as a Source Data file. Full size image We next investigated whether our activators directly interact to Sa ClpP in staphylococcal cells by performing the cellular thermal shift assay (CETSA). We observed significantly increased thermal stability of Sa ClpP when the S. aureus 8325-4 strain was cultured with 10 μM ( R )- or ( S )-ZG197 (Fig. 3d and Supplementary Fig. 3c ). Similar elevation of Sa ClpP T m occurred when bacterial cells were treated with ONC212. This indicates that our selective activators and the global activator ONC212 can directly bind to the Sa ClpP protease in staphylococcal cells. We also performed CETSA in HEK 293T/17 cell line to test whether our activators bind to Hs ClpP. Similar to DMSO, ( R )- and ( S )-ZG197 have minimal effects on the thermal stability of Hs ClpP in HEK 293 T/17 cells, while ONC212 significantly increased Hs ClpP stability (Fig. 3e and Supplementary Fig. 3d ). Therefore, the results in cellular binding assay highlight direct and selective interactions of our activators towards Sa ClpP but not Hs ClpP in cellular contexts, which is similar to the results from the in vitro biophysical binding assays. Identification of critical residues/motif responsible for our activators’ selective binding and activation of Sa ClpP but not Hs ClpP To reveal the structural insight into the mechanism of ( R )- and ( S )-ZG197’ selective activation on Sa ClpP proteolysis, we determined the X-ray crystal structures of ( R )-ZG197/ Sa ClpP ( 7XBZ in PDB) and ( S )-ZG197/ Sa ClpP ( 7WGS in PDB) complexes to a resolution of 2.15 Å and 2.11 Å, respectively (Supplementary Table 1 ). The resolved structures demonstrate that twelve ( R )-ZG197 or fourteen ( S )-ZG197 activators bind in the fourteen hydrophobic pockets of Sa ClpP (Supplementary Fig. 4a ), and the electron density maps distinctly show the existence of ( R )- and ( S )-ZG197, respectively (Fig. 4a, b ). The naphthyl motifs of ( R )- and ( S )-ZG197 point in different directions due to the chiral methyl substituents. The carbonyl group in both ( R )- and ( S )-ZG197 forms a hydrogen bond with H83 of Sa ClpP, and the side chain of Q52 also forms a hydrogen bond with ( R )-ZG197 directly or ( S )-ZG197 mediated by a water molecule. Additional hydrogen bonds mediated by the side chains of D27, L49 jointly contribute to ( S )-ZG197 binding to Sa ClpP (Fig. 4a, b ). In addition, extensive hydrophobic interactions are observed on ( R )- and ( S )-ZG197 in ligand binding sites of Sa ClpP (Supplementary Fig. 4b ). Structural alignment of Sa ClpP ( 6TTY in PDB), ADEP 4/ Sa ClpP ( 6TTZ in PDB), ( R )-ZG197/ Sa ClpP ( 7XBZ in PDB) and ( S )-ZG197/ Sa ClpP ( 7WGS in PDB) yield low Cα root mean square deviation (RMSD) values around 0.2 Å for ClpP monomer, indicating a high similarity of ClpP folding (Supplementary Fig. 4c ) [43] , [46] , [47] . Like the global activator ADEP 4, ( R )- and ( S )-ZG197 bindings induce an extended state of Sa ClpP, which has been characterized by a straight orientation of the α5 helix [26] . Moreover, the catalytic triad (S98, H123 and D172) are also displayed in highly similar orientations in these structures (Supplementary Fig. 4d ). Interestingly, only four or five out of the fourteen N-terminal loops are ordered in the structural complexes of ( R )- and ( S )-ZG197/ Sa ClpP, implying the highly dynamic nature of these motifs upon activators binding. Fig. 4: Identification of key sites/motif for selective Sa ClpP over Hs ClpP activation. Close view of interactions of ( R )- ( a ) and ( S )-ZG197 ( b ) in the hydrophobic site of Sa ClpP. The fo-fc omit map for showing ( R )- and ( S )-ZG197 binding is contoured at 3.0 Å and colored in green, while the 2fo-fc map is contoured at 1.0 Å and colored in magenta, respectively. ( R )- and ( S )-ZG197 are colored in light pink and light blue, respectively. Hydrogen bonds are indicated by dark dashed lines, and the distance is labeled in Å. c Close view of structural alignments of ( R )- and ( S )-ZG197 bound to Sa ClpP complexes, and ZG180 bound to Hs ClpP in the hydrophobic pockets. ZG180, ( R )- and ( S )-ZG197 are colored in cyan, light pink, and light blue, respectively. Sa ClpP is colored in gray, while Hs ClpP is colored in wheat. d Quantitation of α-casein hydrolysis by the Sa ClpPI91W mutant in the presence of ( R )-ZG197, ( S )-ZG197, and ONC212, respectively. e Effect of activators on the thermal stability of the Sa ClpPI91W protein detected in the DSF assay. f Representative Western blot images showing the effects of 10 μM activators on the thermal denaturation of the Sa ClpPI91W protein in intact cells of the complemented clpPI91W mutant strain. Sa ClpPI91W expression was induced in the presence of anhydrous tetracycline (ATC) at 1 ng/mL. Three biological replicates were performed for each experiment. g Quantitation of ClpP activators-promoted hydrolysis of α-casein by the Hs ClpPW146A mutant. h Effect of activators on the thermal stability of the Hs ClpPW146A mutant detected in the DSF assay. i Close view of the structural alignment in ( c ) shows the effect of the C-terminal residues on activators’ binding and activation of Hs ClpP. j Quantitation of effect of activators-activated α-casein hydrolysis by the Hs ClpPΔC (left) and Hs ClpPW146AΔC (right) truncations, respectively. k Effect of activators on the thermal stability of the Hs ClpPΔC (left) and Hs ClpPW146AΔC (right) detected in the DSF assay Data ( d , e , g , h , j , and k ) are obtained from three biologically independent experiments and presented as mean ± SD (error bars). Source data are provided as a Source Data file. Full size image To understand the structural mechanism that causes ( R )- and ( S )-ZG197 to selectively bind to and activate Sa ClpP but not Hs ClpP, we aligned our resolved structures of ( R )-ZG197/ Sa ClpP and ( S )-ZG197/ Sa ClpP to the ZG180/ Hs ClpP structure. The naphthyl group in ( S )-ZG197 is positioned in the opposite direction compared to that in ZG180 and ( R )-ZG197, which results in a direct clash with the side chain of W146 in Hs ClpP. This can restrict ( S )-ZG197 to bind to Hs ClpP in a mode similar to Sa ClpP (Fig. 4c ). While though the naphthyl group in ( R )-ZG197 is positioned away from the side chain of W146 in Hs ClpP, the methyl substituent in ( R )-ZG197 can generate a spatial hindrance and clash with W146 in Hs ClpP, which likely explain why ( R )-ZG197 cannot interact with Hs ClpP. The structural alignment analysis suggests that I91 in Sa ClpP and W146 in Hs ClpP are primarily critical sites responsible for our activators’ selective binding and activating on Sa ClpP but not Hs ClpP. To illustrate how I91 influences our activators’ binding to Sa ClpP, we constructed an I91W mutant in Sa ClpP to mimic the corresponding W146 in Hs ClpP and determined whether ( R )- and ( S )-ZG197 bind to and activate the Sa ClpPI91W mutant. As predicted, ( S )-ZG197 exhibits a significantly diminished activity on the Sa ClpPI91W mutant for α-casein hydrolysis, while ( R )-ZG197 and ONC212 still activate Sa ClpPI91W to degrade α-casein in vitro (Fig. 4d and Supplementary Fig. 4e ). We next investigated the interactions between ClpP activators and the Sa ClpPI91W mutant in DSF. Consistent with the biochemical observation, ( S )-ZG197 cannot thermally stabilize the Sa ClpPI91W mutant, while ( R )-ZG197 and ONC212 still significantly increase the T m of the Sa ClpPI91W mutant (Fig. 4e ). We then quantitatively determined the affinity of ( R )-ZG197 for binding to Sa ClpPI91W, and the K d is 0.93 ± 0.2 μM in ITC assay. No binding was observed between ( S )-ZG197 and Sa ClpPI91W (Supplementary Fig. 4f ). It should be noticed that ( R )-ZG197 is still positive on the Sa ClpPI91W mutant. This is because of the methyl substituent in ( R )-ZG197 that can contribute hydrophobic affinity with W91 in the Sa ClpPI91W mutant, while it likely clashes with W146 in Hs ClpP (Fig. 4c ). A resolved structure of ( R )-ZG197/ Sa ClpPI91W complex would be beneficial for revealing the mechanism of this phenomenon. In addition, we constructed the complemented clpPI91W mutant strain via a tetracycline-inducible expression vector pYJ335 in the Δ clpP mutant (Supplementary Fig. 4g ), and assessed the cellular interactions between the activators and the Sa ClpPI91W mutant in the complemented strain. In line with the observed interactions in vitro, ( S )-ZG197 treatment fails to induce the T m shift of Sa ClpPI91W in intact staphylococcal cells, while ( R )-ZG197 and the global activator ONC212 exhibit strong effects on Sa ClpPI91W stabilization (Fig. 4f and Supplementary Fig. 4h ). We also constructed the Hs ClpPW146A mutant to test whether the proposed steric clash between our activators and the rigid side chain of W146 restricts their binding to Hs ClpP. In contrast to the observation that ( R )-ZG197 is inactive on Hs ClpP, ( R )-ZG197 becomes active to promote the Hs ClpPW146A mutant for α-casein hydrolysis (Fig. 4g and Supplementary Fig. 4i ), and displays binding affinity towards Hs ClpPW146A as measured in DSF assay (Fig. 4h ). ONC212 always binds to and activates both Hs ClpP and the W146A mutant in vitro. However, since ( S )-ZG197 fails to bind to and activate Hs ClpPW146A, we hypothesized that other structural factors attenuate the interaction of ( S )-ZG197 and Hs ClpP mutant. Previously, it was suggested that the extra motif in the Hs ClpP C-terminus disturbs the ClpX chaperone’s binding [48] . Particularly, we noticed the P248 and P249 residues might form a lid motif that could hinder activators’ approaching and binding to the hydrophobic sites of Hs ClpP (Fig. 4i ). This extra lid motif in Hs ClpP is also conserved in other eukaryotic ClpPs, like Mus Musculus ClpP ( Mo ClpP) and Danio Rerio ClpP ( Da ClpP). However, this C-terminal sequence is shortened and the corresponding lid motif is absent in the bacterial ClpPs, such as Sa ClpP and Escherichia coli ClpP ( Ec ClpP) (Supplementary Fig. 2a ). We then purified the C-terminal truncated Hs ClpP ( Hs ClpPΔC) and Hs ClpPW146A ( Hs ClpPW146AΔC) proteins and detected our activators’ effects on the two truncations. Similar to the weak effects on Hs ClpPW146A, ( S )-ZG197 still minimally activates and barely stabilizes Hs ClpPΔC in vitro (Fig. 4j and k and Supplementary Fig. 4j ). However, ( S )-ZG197 becomes active to promote Hs ClpPW146AΔC mutant for α-casein hydrolysis and displays binding affinity as measured in DSF (Fig. 4j and k and Supplementary Fig. 4k ), indicating the joint action of W146 and C-terminal motif in Hs ClpP. Interestingly, both ( R )-ZG197 and ONC212 exhibit improved capabilities for binding to and activating on Hs ClpPW146AΔC compared to Hs ClpPW146A and Hs ClpPΔC (Fig. 4j and k and Supplementary Fig. 4k ). Altogether, this indicates that the two distinct amino acids (I91 in Sa ClpP and W146 in Hs ClpP) in the hydrophobic pockets and the extra C-terminal lid motif in Hs ClpP are crucial factors that can determine the selective activation of Sa ClpP over Hs ClpP by our species-specific activators. Our activators exhibit antibacterial activity in a Sa ClpP-dependent manner We next performed a minimum inhibitory concentration (MIC) assay in liquid culture to determine the antibacterial effects of our activators on the S. aureus 8325-4 strain. ( R )-ZG197 significantly suppresses S. aureus with a quantified MIC of 0.5 μg/mL, which is as active as ONC212 (Fig. 5a ). ( S )-ZG197 also inhibits the growth of S. aureus 8325-4, and the MIC is 4 μg/mL. Both ( R )-ZG197 and ( S )-ZG197 exhibit much better inhibitory effects on staphylococcal growth than the hit compound ICG-001. To dissect whether our activators’ antistaphylococcal activity depends on ClpP in S. aureus , we determined the inhibitory effects of our activators on the Δ clpP mutant and the complemented clpP or clpPI91W mutant strains, respectively (Fig. 5a ). The selective ( R )- and ( S )-ZG197 activators or the global activators ICG-001 and ONC212 minimally suppress the growth of Δ clpP mutant strain, and all the MICs are observed to be over 256 μg/mL. The antibacterial phenotype can be rescued in the complemented clpP strain in the presence of ClpP activators. Unlike ( R )-ZG197 and ICG-001 and ONC212, the antibacterial activity of ( S )-ZG197 is significantly attenuated in the complemented clpPI91W mutant strain since ( S )-ZG197 is inactive on the Sa ClpPI91W mutant in vitro and in cells. This indicates that our activators exhibited antibacterial activities in a Sa ClpP-dependent manner in S. aureus . Fig. 5: Target dependency of ( R )- and ( S )-ZG197’ antibacterial activity in cellular contexts. a Assessment of ClpP activators on the growth of S. aureus 8325-4 with genetic backgrounds of clpP , Δ clpP , and complemented clpP or I91W mutant by MIC measurement. b Assessment of Sa ClpP activators’ effect on the cellular Sa FtsZ abundance in the intact cells of 8325-4, Δ clpP , the complemented clpP and clpPI91W strains detected in Western blot. Quantitation on the band intensity of Sa FtsZ is normalized against the loading control of Sa GAPDH, and the ratio in the DMSO group is considered as 1.0. c Representative views of SEM micrographs showing the effects of ( R )- and ( S )-ZG197 on the cell morphology of S. aureus 8325-4 having different genetic backgrounds of clpP , Δ clpP , and complemented clpP or clpPI91W . The scale bar represents 1 μm. d Representative views of SEM micrographs showing the effect of 20 µM ( R )- and ( S )-ZG197 on cell division of Newman and USA300 strains. The scale bar represents 1 μm. e Determination of MIC of the Sa ClpP activators against the growth of a panel of S. aureus strains. ( R )- and ( S )-ZG197, ONC212, and the clinic antibiotics oxacillin, tetracycline, erythromycin, norfloxacin, clindamycin, and gentamicin were assayed under similar conditions. The experiments were performed in triplicates. f Bactericidal effect of ( R )- and ( S )-ZG197 combined therapy on eradicating stationary phase USA300 ( n = 3 biologically independent experiments). Cell numbers were recorded in CFU/mL. Data are presented as mean ± SD. Source data are provided as a Source Data file. Full size image The cell division protein Sa FtsZ could be over-degraded upon the aberrant activation of Sa ClpP in the presence of activators in cells [25] . Indeed, all activators, including ( R )-ZG197, ( S )-ZG197, and ONC212, decrease Sa FtsZ abundance in the 8325-4 S. aureus but not in the corresponding Δ clpP mutant strain, as detected by the immunoblotting assay (Fig. 5b ). The Sa FtsZ abundances are dramatically decreased in the complemented clpP or clpPI91W mutant in the presence of the selective activator ( R )-ZG197 or the global activator ONC212. Similar to the observation that ( S )-ZG197 could not activate the Sa ClpPI91W mutant protease activity, we observed no obvious decrease in the abundance of Sa FtsZ in the complemented clpPI91W strain in the presence of ( S )-ZG197. This indicates that our activators induced the aberrant degradation of Sa FtsZ in S. aureus , which is highly dependent on the cellular Sa ClpP. The dysregulated degradation of Sa FtsZ could impair cell division in S. aureus [24] , [25] . We then measured the cell morphology of staphylococcal cells using a scanning electron microscope (SEM), which could reflect the inhibitory effects of our activators on staphylococcal cell division [49] . The diameters of staphylococcal cells are measured as 0.64 μm, 0.69 μm, 0.73 μm, and 0.75 μm in average for 8325-4, Δ clpP , and complemented clpP or clpPI91W strains in vehicle groups, respectively (Fig. 5c and Supplementary Fig. 5a ). Interestingly, similar to the inhibitory effects of FtsZ inhibitor TXA709 on staphylococcal cell division, ( R )- and ( S )-ZG197 treatments significantly enlarge the cell diameters of 8325-4 and the complemented clpP strains, with the measured diameters usually larger than 1.00 μm [50] . Shrinking, lysis, and full degradation of staphylococcal cell morphology were observed in bacteria treated with our activators. In contrast, we did not observe changes in the bacterial diameter or cell morphology when the Δ clpP mutant was exposed to ( R )- and ( S )-ZG197 activators. Treatment with ( R )-ZG197 results in enlarged cells size in the complemented clpPI91W mutant strain, while ( S )-ZG197 has no effect on bacterial diameter in this strain. 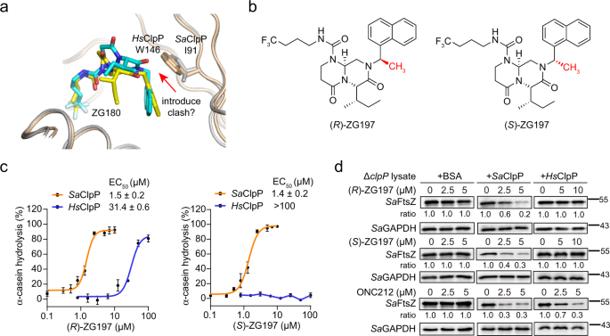Fig. 2: Design and development of selectiveSaClpP activators. aStructural superimposition of ZG180/SaClpP and ZG180/HsClpP complexes to reveal the strategy for designing selective activators forSaClpP overHsClpP.SaClpP andHsClpP are shown in gray and wheat cartoon tubes, respectively. ZG180 is colored in cyan in the ZG180/SaClpP structure, while it is colored in yellow in the ZG180/HsClpP structure. I91 inSaClpP and W146 inHsClpP are shown as a stick.bStructures ofSaClpP activators (R)- and (S)-ZG197 developed by the structure-based design outlined in (a). The chiral methyl group is indicated in red.cQuantitation of α-casein hydrolysis bySaClpP andHsClpP in the presence of (R)- and (S)-ZG197, respectively (n= 3 biologically independent experiments). Data are presented as mean ± SD (error bars).dEffect of activators on degradation of the cellularSaFtsZ protein with the supplement of bovine serum albumin (BSA), the recombinantSaClpP, andHsClpP, respectively, in cell lysates of theclpPdeletion (ΔclpP) mutant. The abundance of cellularSaFtsZ is quantitated with a Western blot assay. Quantitation on the band intensity ofSaFtsZ is normalized against the loading control ofSaGAPDH, and the ratio in the DMSO group is considered as 1.0. Source data are provided as a Source Data file. We also tested the effect of our selective activators on cell divisions in Newman, a clinical isolate of methicillin-sensitive S. aureus strain, and in USA300, a representative MRSA isolate (Supplementary Table 2 ). A similar phenomenon of enlarged diameters in Newman and USA300 cells was observed in the presence of ( R )- and ( S )-ZG197 (Fig. 5d , Supplementary Fig. 5b, c ). We demonstrated that ( R )- and ( S )-ZG197 exhibit suppressive effects on cell division in S. aureus , which is dependent on the cellular Sa ClpP. Given our species-specific activators suppress the growth of S. aureus 8325-4, we then tested the antistaphylococcal spectrum of ( R )- and ( S )-ZG197 against a panel of S. aureus strains, including the Newman strain and multidrug-resistant MRSA strains. The USA300, NRS-1, NRS-70, NRS-100, NRS-108, and NRS-271 MRSA strains were collected from the Network on Antimicrobial Resistance in S. aureus (Supplementary Table 2 ). ( R )-ZG197 displays strong antibacterial activity on a broad spectrum of these S. aureus strains, with MIC values of 0.5-2 μg/mL, while ( S )-ZG197 suppresses the growth of these strains with moderate MIC values of 2–8 μg/mL (Fig. 5e , left panel). We also tested the antibacterial effects of our activators on five hospital-acquired, multidrug-resistant MRSA isolates in China, including XJ009, XJ036, XJ049, XJ051, and XJ052 (Supplementary Table 2 ). These clinical MRSA isolates have developed remarkable resistance towards several clinical antibiotics, including oxacillin, tetracycline, erythromycin, norfloxacin, clindamycin, and gentamicin, but they are all sensitive to our activators with MIC values of 0.5-1 μg/mL for ( R )-ZG197 and 2–8 μg/mL for ( S )-ZG197, respectively (Fig. 5e , right panel). The global activator ONC212 also exhibits low MIC values on these strains. Similar to ONC212 and vancomycin, both ( R )-ZG197 and ( S )-ZG197 exhibit excellent bactericidal effects on the exponentially growing Newman strain (Supplementary Fig. 5d ). We next assessed the antibacterial effects of our activators on eradicating persisters, which are cells subjected to acute stress to arouse antibiotic persistence [51] . A cohort of overnight stationary phase S. aureus cells that suffered from nutrient limitation are persisters and were difficult to be eradicated with conventional antibiotics [52] . Like the well-established ClpP activator ADEPs, ( R )-ZG197, ( S )-ZG197, rifampicin, and ciprofloxacin each alone minimally reduce the colony-forming units (CFU) of the MRSA strain of USA300 cultures (Fig. 5f and Supplementary Fig. 5e ), while a combined therapy using either ( R )-ZG197 or ( S )-ZG197 with rifampicin or ciprofloxacin significantly reduces the number of USA300 persisters to the limit of detection (Fig. 5f ). To further investigate the suppressive effect of combined therapy on persistent S. aureus cells, we performed a biphasic killing assay on the USA300 strain. Similar to ADEP 4 [23] , we found that adding a second conventional antibiotic, such as rifampicin or ciprofloxacin, slightly impair the growth of ciprofloxacin-induced persisters, while the presence of ( R )- and ( S )-ZG197 Sa ClpP activators completely eradicate persisters to the limit of detection (Supplementary Fig. 5f ). Collectively, these results verify that our activators eradicate staphylococcal persisters as efficiently as ADEP 4 when combined with conventional antibiotics. We also screened the resistant mutants of Sa ClpP induced by our species-specific activators. Resistance rates are defined according to the established protocol [47] . The frequencies of spontaneous resistance induced by 4 × MIC of ( R )-ZG197 and ( S )-ZG197 are in the range of 10 −7 , which are comparable with ADEP 4 and ONC212, the global activators of ClpP. 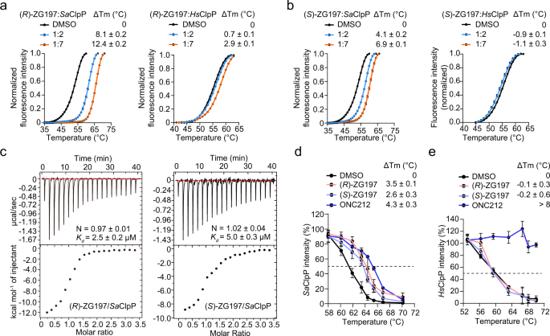Fig. 3: Investigation of the interaction between species-selective activators andSaClpP. Effect of (R)- (a) and (S)-ZG197 (b) on the thermal stability ofSaClpP andHsClpP in DSF assay, respectively. Tm, melting temperature.cDetermination of (R)- and (S)-ZG197 binding toSaClpP by ITC titration. The dissociation constant (Kd) and stoichiometry factor (N) are indicated. Effect of activators on the thermal stability of the cellularSaClpP (d) andHsClpP (e), respectively. TheS. aureus8325-4 was cultured in the presence of 10 μM compound for 2 h before running CETSA (d), while cell lysates of HEK 293 T/17 were assayed in CETSA (e). The proteins in unheated samples are used as inputs and considered as 100%. Data (a,b,d, ande) are obtained from three biologically independent experiments and presented as mean ± SD (error bars). Source data are provided as a Source Data file. All mutation sites are randomly distributed and located outside of the hydrophobic binding pockets of ClpP (Supplementary Table 3 ). Anti-infective effects of ( R )- and ( S )-ZG197 in vivo To test the anti-infective effects of our activators in vivo, we first assessed their bioactive profiles. Unlike the screening hit compound ICG-001 that was initially identified as a Wnt/β-catenin inhibitor, ( R )- and ( S )-ZG197 minimally disrupt the Wnt/β-catenin signaling pathway in HEK 293T/17 and HK-2 cell lines in the Wnt/β-catenin luciferase reporter assay (Supplementary Fig. 6a ) [39] . We then investigated the effects of our Sa ClpP activators on viability of HEK 293T/17 and HK-2 cell lines in MTT assay. As anticipated, ( R )- and ( S )-ZG197 have minimal toxic effects on proliferation of mammalian cells, as evidenced by low inhibitory activities with high IC 50 values (Supplementary Fig. 6b ). In contrast, the global activator ONC212 and our hit compound ICG-001 dramatically inhibit mammalian cell viability, especially ONC212, which has low IC 50 values of 20–60 nM. We also assessed the cytotoxic effect of our activators on zebrafish. The administration of ( R )- or ( S )-ZG197 at a single dose of 25 or 50 mg/kg has no cytotoxic effect on zebrafish survival (Supplementary Fig. 6c ). When administrated at 100 mg/kg, ONC212 significantly cause zebrafish death, while ( R )- or ( S )-ZG197 is still safe on zebrafish (Supplementary Fig. 6c ). This indicates the biosafety of our species-specific activators for antistaphylococcal infections in vivo. We then evaluated the in vivo antibacterial effects of ZG197 using a zebrafish infection model, which is a widely used in vivo model for assessing antistaphylococcal agents against S. aureus infections [53] . We first determined an appropriate CFUs of S. aureus that can lead to zebrafish mortality within a reasonable time window (Supplementary Fig. 6d ). We evaluated the antibacterial potency of our Sa ClpP activators by measuring the survival rate of zebrafish after a staphylococcal infection for five days (Supplementary Fig. 6e ). A single administration of 50 mg/kg of ( R )- and ( S )-ZG197 significantly prolong the survival rate of USA300-infected zebrafish (Fig. 6a ). A lower dose of ( R )- or ( S )-ZG197 at 25 mg/kg also effectively protect zebrafish against USA300-induced lethal infection (Supplementary Fig. 6f ). Similarly, the administration of 25 mg/kg or 50 mg/kg ( R )-ZG197 effectively improve the survival rate of Newman-infected zebrafish, which has a better survival rate than ONC212 (Supplementary Fig. 6g and Fig. 6b ). However, ( R )-ZG197 loses therapeutic effects on zebrafish infected with the Δ clpP mutant strain, while vancomycin is still active against this infection (Fig. 6c ). This indicates that the promising antistaphylococcal effect of ( R )-ZG197 on infected zebrafish is dependent on Sa ClpP in vivo. A single administration of 50 mg/kg of ( R )-ZG197 produce a significant therapeutic effect on zebrafish infected with the clinical MRSA strain XJ049. In contrast, this strain is resistant to the treatment of clinically used antibiotics oxacillin and erythromycin (Fig. 6d ). It is unsurprising that the global activator ONC212 at 50 mg/kg fail to prolong the survival rate of zebrafish infected with MRSA XJ049 likely due to its cytotoxic side-effects by targeting Da ClpP (Fig. 6d ). Fig. 6: Anti-infective effects of ( R )- and ( S )-ZG197 in vivo. a Therapeutic effect of ( R )- and ( S )-ZG197 against USA300 infection in zebrafish. Zebrafish ( n = 11 animals) were infected with 7 × 10 6 CFU of USA300, and compounds were administered at a single dose of 50 mg/kg. DMSO (5%) and vancomycin were administered as controls. Therapeutic effect of ( R )-ZG197 against lethal infection by Newman ( b ) and the Δ clpP mutant ( c ). Zebrafish ( n = 11 animals) were infected with 7 × 10 7 CFU of Newman ( b ) or 3 × 10 7 CFU of the Δ clpP mutant ( c ), and compounds were administered to infected zebrafish at 50 mg/kg. Vancomycin and ONC212 were used as controls. d Therapeutic effect of ( R )-ZG197 on the clinical MRSA isolates infected zebrafish. Zebrafish ( n = 11 animals) were infected with 5 × 10 7 CFU of XJ049, and compounds were administered at a single dose of 50 mg/kg. DMSO (5%), antibiotics (vancomycin, erythromycin, and oxacillin), and the global activator ONC212 were used as controls. e Quantitation of necrotic skin lesion size of initial (left panel) and 4 days post-infection (right panel). Vancomycin was used as a positive control. Data are shown as mean ± SD ( n = 9 animals). f Representative images showing necrotic skin lesions 4 days post-infection. The scale bar represents 1 cm. g Effects of our activators on bacterial counts in the skin samples ( n = 8 biologically independent samples). Skin tissue was excised from mice infected with USA300 4 days post-infection and plated onto TSA to enumerate CFUs. h Micrographs of H&E-stained skin tissues after the indicated treatments. The scale bar represents 1 mm (Top) and 0.1 mm (Bottom). Statistical differences were analyzed using Log-rank tests ( a – d ) and two-tailed unpaired Student’s t -tests ( e , g ). Exact P values are provided. ns, no significance. Data ( e , g ) are presented as mean ± SD (error bars). Source data are provided as a Source Data file. Full size image Lastly, we evaluated the in vivo anti-infective efficacy of our activators in murine skin S. aureus infection models [54] . Mice skin was inoculated with 2.5 × 10 6 CFUs of USA300 and a lesion appeared after 16 h. The initial lesion areas in each group are comparable (Fig. 6e ). Subcutaneous injection of ( R )- and ( S )-ZG197 at 7.5 mg/kg twice a day causes a smaller necrotic lesion size in mice compared with the vehicle control (Figs. 6 e, f ). Moreover, we observed a significant reduction in bacterial load when we excised the lesions of mice treated with ( R )- and ( S )-ZG197 compared to the vehicle control (Fig. 6g ). Histological analysis using hematoxylin and eosin (H&E) staining also exhibits a decrease in the necrotic area and inflammatory infiltrates in the skin tissues when treated with our activators or vancomycin, while the vehicle-treated sample displays dense inflammatory infiltrates (Fig. 6h ). Collectively, we identify our activators as promising antibiotics against multidrug-resistant MRSA infections in vivo but with minimal cytotoxic effects. Aberrant activation of bacterial ClpP protease is a promising method of treating nosocomial infections with antibiotic-resistant Gram-positive bacteria. The desired Sa ClpP activator should preferably target the staphylococcal ClpP rather than disturb the proper function of the host ClpP. However, earlier work identified several global activators for the ClpP proteases of multiple species, including ADEP analogs and ONC212, which would inevitably produce unintended off-target effects and hamper the application in drug discovery for anti-MRSA infection. Therefore, identifying distinct chemical scaffolds that selectively activate Sa ClpP will highlight its anti-infective therapeutic potential for MRSA infections using a chemoactivation strategy. We use HTS for compounds that promote the ClpP protease activity and experimental validation to identify N -benzyl- and naphthalen-1-ylmethyl-disubstituted peptidomimetic compound (ICG-001) as an activator with a moderate activity for both Sa ClpP and Hs ClpP. Synthetic optimization of ICG-001 analogues led to discovery of (6 S ,9a S )-6-(( S )-sec-butyl)-8-(naphthalen-1-ylmethyl)-4,7-dioxo- N -(4,4,4-trifluorobutyl)hexahydro-2 H -pyrazino[1,2-a]pyrimidine-1(6 H )-carboxamide (ZG180) with significantly improved activities on both proteases. The incorporation of methyl substituent group on ZG180 makes ( R )- and ( S )-ZG197 the most potent and highly selective activators for Sa ClpP over Hs ClpP. Our activators increase the aberrant degradation of Sa FtsZ protein in cells, inhibit staphylococcal cells division, and display significant antibiotic efficacy in preventing the lethal outcome of S. aureus bacteremia in vivo. Earlier work demonstrated ICG-001 as an inhibitor for the Wnt/β-catenin signaling pathway and exerted antiproliferative effects in xenografted murine models. Nevertheless, our activators minimally inhibit the viability of mammalian cell lines, which should be explored further during the clinical development of antibiotics. Our identification of ( R )- and ( S )-ZG197 as species-specific activators for Sa ClpP provides structural insights into the development of selective binding and specific chemoactivation of certain ClpP. The bulky W146 of Hs ClpP affords an unfavorable steric clash with the hindrance naphthyl substituent in ( S )-ZG197 activator, therefore prevents ligands’ binding to Hs ClpP. This indicates W146/I91 residue is a critical factor that partially determines the species-selectivity of our activators. In addition to the observation that W146 in Hs ClpP represents a critical point for activator discrimination, our work also reveals W146’s joint action with the C-terminal motif in Hs ClpP, as evidenced by the recovered activities of ( S )-ZG197 and the improved activities of ( R )-ZG197 towards Hs ClpPW146AΔC’s binding and activation compared to either the Hs ClpPW146A mutant or the Hs ClpPΔC truncation. Along with previously published research, this shows that the key structural factors, including spatial difference in hydrophobic pockets and coordination of other amino acids, significantly contribute to the discrimination of ClpP activators. Additionally, variant activators respond differently to the bacterial and mitochondrial ClpP proteins. Chemoactivation of bacterial ClpP efficiently switches it into an uncontrollable state to trigger excessive degradation of numerous substrates that are crucial to bacteria and ultimately destroy the pathogenic bacteria. We demonstrate that both ( R )-ZG197 and ( S )-ZG197 selectively bind to Sa ClpP over Hs ClpP, induce the activator-bound Sa ClpP in the fully extended, active conformation for nonselective hydrolysis of essential proteins, such as FtsZ. Although bacterial ClpP is not essential for survival, the ClpP activators are inclined to induce ClpP mutation and thus develop resistance. Therefore, combination therapy is likely the best method of therapeutic application for Sa ClpP activators, which could lower target-based resistance, broaden the antibiotic spectrum, and reduce dosage and unwanted side-effects. We also show that either ( R )-ZG197 or ( S )-ZG197 used in combination with rifampin or ciprofloxacin dramatically eradicates the population of persisters to the detection level. Given highly conserved ClpP proteases among multiple species, it must be investigated whether our activators can similarly switch other ClpP proteases from different species into gain-of-function states, especially with Gram-negative bacteria and gut microbiota. Further synthetic optimizations are needed to improve the antimicrobic capabilities of our species-specific Sa ClpP activators to treat MRSA infections. Assessment of the anti-infective effects of our activators on additional in vivo animal infectious models would fully characterize the antibacterial potency of these activators. In conclusion, we report ( R )- and ( S )-ZG197 as selective Sa ClpP activators and identify the critical residues/motif for selectively promoting Sa ClpP rather than Hs ClpP. Our data provide mechanistic insights into the chemoactivation of ClpP proteases and accelerate the discovery of species-specific antibiotic drugs that can selectively disturb the function of staphylococcal protease. This work has the potential to inspire promising strategies for treating MRSA infections and contributes to the generation of potent synthetic antibiotic scaffolds with minimal cytotoxicity to the host. Animals Wild-type zebrafish (7 to 11 months old, 300 ± 50 mg, regardless of gender) were purchased from the Xiaoguan aquarium (Shanghai, China) and maintained in a 10-L tank at ambient temperature with regular feeding. Similar size and random sex distribution of zebrafish were used for S. aureus infection. Female BALB/c mice (6 to 8 weeks old, 18–20 g) were purchased from Zhejiang Vital River Laboratory Animal Technology Co., Ltd. All mice were housed on an ad libitum diet in the specific pathogen-free facility at Shanghai Public Health Clinical Center. Housing conditions of dark/light cycle 12 h, ambient temperature 20–26 °C, humidity 40–60% were applied on mice. Antibodies Antibodies of Sa ClpP (1:5,000, Cat#C11185), Sa FtsZ (1:5,000, Cat#C11186), and Sa GAPDH (1:5,000, Cat#C1399) were generated by Shanghai Immune Biotech Ltd using the purified protein as the antigen and validated by ELISA experiments. Antibodies of Hs ClpP (1:2,000, Clo#EPR7133, Cat#ab124822, Lot#GR3210822-8, Abcam), β-actin (1:5,000, Clo#2D4H5, Cat#66009-1-Ig, Lot#10004156, Proteintech), HRP-conjugated goat anti-rabbit IgG (1:10,000, Cat#CW0103, Cwbio), and HRP-conjugated goat anti-mouse IgG (1:10,000, Cat#CW0102, Cwbio) were commercially purchased. Bacterial strains and mediums The bacterial strains used in this study are provided in Supplementary Table 2 . Mediums of Tryptic Soy Broth (TSB, OXOID), Tryptone Soya Agar (TSA, OXOID), Brian Heart Infusion (BHI, OXOID), Mueller-Hinton agar (MHA, Dalian Meilun Biotech) and Mueller-Hinton Broth (MHB, Dalian Meilun Biotech) mediums were used for cultivation of S. aureus . Luria Bertani (LB) in broth or LB agar mediums were used for Escherichia coli ( E. coli ) growth. Chemicals ZG180, ( R )- and ( S )-ZG197 were synthesized in lab and fully characterized. ONC212 and ADEP 4 were purchased from Topscience and ChemPartner (Shanghai, China), respectively. Antibiotics of vancomycin, spectinomycin, erythromycin, ciprofloxacin, rifampicin, tetracycline, norfloxacin, clindamycin, and gentamicin, were purchased from Dalian Meilun Biotech. Oxacillin was purchased from Sigma-Aldrich. Anhydrous tetracycline (ATC) was purchased from APExBIO. Mammalian cell lines and cultures The HEK 293T/17 (CRL-11268) and HK-2 (CRL-2190) cell lines were purchased from the American Type Culture Collection (ATCC). Cells were cultured in Dulbecco’s Modified Eagle Medium (DMEM, Corning) supplemented with 10% fetal bovine serum (FBS, GIBCO) and 1% penicillin-streptomycin (Corning). Cells were cultured at 37 °C in a humidified, 5% CO 2 -containing atmosphere incubator (Thermo Scientific). All cells have been validated by short tandem repeat (STR) profiling and were regularly checked to be mycoplasma-free. Cloning and protein purification The plasmid pET28b -Sa ClpP was used for Sa ClpP expression [49] . E. coli BL21 (DE3) Gold strains were transformed with the plasmid in the presence of 30 μg/mL kanamycin. When OD 600 (absorbance at the wavelength of 600 nm) reaches 0.6-0.8, protein expression was induced by 0.5 mM Isopropyl β-D-1-thiogalactopyranoside (IPTG) at 30 °C for 4 h. Then cell pellets were harvested and stored at −80 °C. Cells were lysed and the supernatant was subjected to 5 mL HisTrap TM HP (GE Healthcare) column in binding buffer (50 mM Tris-HCl, pH 8.0, 100 mM NaCl, and 50 mM imidazole), and then eluted with elution buffer (50 mM Tris-HCl, pH 8.0, 100 mM NaCl, and 400 mM imidazole). The eluted proteins were concentrated with Amicon Ultra Centrifugal Filters with 10 kDa cutoff (Merck-Millipore) and subjected to gel filtration on an AKTA purifier system with a HiLoad 16/60 Superdex 200 column (GE Healthcare) in 20 mM HEPES, pH 7.0 and 100 mM NaCl. The site-directed mutation of Sa ClpPI91W was established according to the Quikchang Site-Directed mutagenesis Kit (Stratagene). A similar procedure was applied on Sa ClpPI91W purification. The plasmid pET28a -Sa FtsZ was used for Sa FtsZ expression [49] , and transformed into E. coli BL21 (DE3) Gold in the presence of 30 μg/mL kanamycin. When OD 600 reaches 0.6, expression of Sa FtsZ was induced by 0.5 mM IPTG for 12 h at 16 °C. Then cell pellets were lysed, and the supernatant was bound with 5 mL HisTrap TM HP column in binding buffer (50 mM Tris-HCl, pH 8.0, 200 mM NaCl, and 50 mM imidazole), and then eluted with elution buffer (50 mM Tris-HCl, pH 8.0, 200 mM NaCl, and 400 mM imidazole). The eluted proteins were concentrated with Amicon Ultra Centrifugal Filters with 10 kDa cutoff (Merck-Millipore) and was stored at −80 °C. The pPSUMO- CLPP ΔN56 plasmid was transformed to E. coli Rosetta (DE3) cells for Hs ClpP expression [40] . The cells were cultured at 37 °C until OD 600 reached 0.6-0.8 and the expression of Hs ClpP was induced by 0.5 mM IPTG at 37 °C for 4 h. Cells were lysed in binding buffer (20 mM Tris-HCl, pH 7.5, 500 mM NaCl, 10 mM imidazole, and 10% glycerol). The supernatant was then passed through a 5 mL HisTrap TM HP column. After washing with binding buffer, target protein was eluted with elution buffer (20 mM Tris-HCl, pH 7.5, 500 mM NaCl, 500 mM imidazole, and 10% glycerol). The collected protein was then concentrated and resuspended in binding buffer. Then, the ULP1 protease was added to cleave the N-terminal His-SUMO tag at 4 °C overnight with gentle shaking. The remaining fractions were then passed through HisTrap TM HP column for removing the His-SUMO tag and the His-tagged ULP1. Further purification was conducted through a HiLoad 16/60 Superdex 200 column in 20 mM Tris-HCl, pH 7.5, 500 mM NaCl, and 5% glycerol. The construction of plasmids for Hs ClpPW146A, Hs ClpPΔC, and Hs ClpPW146AΔC were performed according to the Quikchang Site-Directed mutagenesis Kit. The purifications of Hs ClpPW146A, Hs ClpPΔC, and Hs ClpPW146AΔC were similar to that of Hs ClpP. The proteins were stocked at −80 °C in 30% glycerol. The primer’s sequences used for constructing plasmids for mutants are shown as follows: SaclpP I91W-F: GATGTTCAAACATGGTGTATCGGTATGGC SaclpP I91W-R: GCCATACCGATACACCATGTTTGAACATC HsCLPP W146A-F: CCGATTTGTACCGCCTGTGTGGGTC HsCLPP W146A-R: GACCCACACAGGCGGTACAAATCGG HsCLPP ΔC-F: GTGCTGGTTCATTAGCCGCAGGATGGTGAAGATG HsCLPP ΔC-R: CATCTTCACCATCCTGCGGCTAATGAACCAGCAC SDS-PAGE based α-casein hydrolysis assay Ten microgram Sa ClpP, Sa ClpPI91W, Hs ClpP or Hs ClpPW146A were dissolved in 50 μL buffer containing 25 mM HEPES-KOH (pH 7.6), 200 mM KCl, 5 mM MgCl 2 , 1 mM EDTA, 10% (v/v) glycerol, and 2 mM DTT, while 10 μg Hs ClpPΔC or Hs ClpPW146AΔC was dissolved in 50 μL buffer containing 25 mM HEPES-KOH (pH 7.6), 5 mM MgCl 2 , 5 mM KCl, 0.03% Tween-20, 10% glycerol, and 2 mM DTT. Various concentrations of compound (final concentration of DMSO at 1%) were preincubated at room temperature for 15 min. Then 0.72 mg/mL α - casein was added, and the reaction was performed at 37 °C for 2 h. The samples were mixed with SDS loading buffer and analyzed by 12% SDS-PAGE followed by Coomassie Brilliant Blue R-250 staining. The EC 50 values were calculated by GraphPad Prism 8 from three biological replicates. High-throughput screening (HTS) for Sa ClpP activators The tetradecameric Sa ClpP protein (0.6 μM) in PD buffer (25 mM HEPES-KOH (pH 7.6), 200 mM KCl, 5 mM MgCl 2 , 1 mM EDTA, 10% (v/v) glycerol, and 2 mM DTT) and compounds (40 μM) were added into the black flat-bottomed 384-well plates. After incubating at 37 °C for 30 min, fluorescence-labeled substrate FITC-casein (0.048 mg/mL) (Sigma) was added, and the hydrolysis reaction was initiated at 37 °C. After 2 h, the fluorescence signals were recorded at the wavelength of 485 nm for excitation and 535 nm for emission using a microplate reader (TECAN). Synthesis and characterization of ZG180 and ( R )- and ( S )-ZG197 ZG180 and ( R )- and ( S )-ZG197 were synthesized in this lab and the synthetic methods along with the characterizations are provided in Supplementary methods and Supplementary Fig. 7 – 23 . Crystallization and structure determination The Sa ClpP and Hs ClpP proteins were crystalized by the sitting drop vapor diffusion method at 16 °C. The sample of 10 mg/mL protein was mixed with 5-fold concentration of the compound of ZG180, ( R )- or ( S )-ZG197 (contain 5% DMSO) and incubated for 30 min at 4 °C. The drops contained 1 or 2 μL Sa ClpP sample and 1 μL reservoir solution of 30%(v/v) 2-methyl-2,4-pentanediol, 0.1 M sodium acetate/HCl (pH 8.0), 20 mM calcium chloride in the presence of ZG180, or 1 μL reservoir solution of 30% v/v (+/−)-2-methyl-2,4-pentanediol, 0.1 M sodium acetate trihydrate (pH 4.6), 200 mM sodium chloride in the presence of ( R )- and ( S )-ZG197. The Hs ClpP sample at 10 mg/mL was incubated in the presence of 5-fold concentration of ZG180 on ice for 30 min and mixed with a reservoir solution of 20% w/v polyethylene glycol 3350, 0.2 M sodium malonate (pH 5.0). These crystals grew up after one week to more than one month. Then the crystals were fished and soaked in 20% (v/v) glycerol for 30 s following with storing in liquid nitrogen. Diffraction data of ZG180/ Sa ClpP and ( R )-ZG197/ Sa ClpP were collected via Bluice at Shanghai Synchrotron Radiation Facility (SSRF) beamline BL19U1 [55] . X-ray data were processed via HKL2000 program suite. Diffraction data of ZG180/ Hs ClpP or ( S )-ZG197/ Sa ClpP were collected via Finback at SSRF beamline BL02U1 and automatically processed by Aquarium [56] . The structures were resolved using the Sa ClpP (PDB code 3STA ) and Hs ClpP (PDB code 1TG6 ) as the search model and models were built in COOT [43] , [48] , [57] . Finally, the data was refined with the program REFMAC5 [58] . The free reflections were automatically selected and applied in all refinements. Structure alignments were performed in PyMOL [59] . In vitro Sa FtsZ degradation assay The Sa FtsZ degradation was analyzed in SDS-PAGE in vitro. Briefly, 10 μg Sa ClpP was dissolved in 50 μL PD buffer. After adding various concentrations of compound (final concentration of DMSO at 1%), the mixture was incubated at room temperature for 15 min. Then Sa FtsZ (1.5 μM) was added, and the reaction was performed at 37 °C for 2 h. The samples were mixed with SDS loading buffer and analyzed by 12% SDS-PAGE followed by Coomassie Brilliant Blue R-250 staining. The EC 50 values were calculated by GraphPad Prism 8 from three biological replicates. The cell lysate of 8325-4/Δ clpP strain was also used in Sa FtsZ degradation assay. An overnight staphylococcal culture of 8325-4/Δ clpP was diluted 1:500 and cultured to early-mid exponential phase (OD 600 = 0.4–0.6) at 37 °C. Culture was then washed with PD buffer for three times followed by cell lysis using 0.75 U Lysostaphin (Sigma). Then the cell lysate was centrifuged at 12,396 × g and the supernatant was collected and divided into 50 μL. Nine micromolar bovine serum albumin (BSA, Dalian Meilun Biotech), Sa ClpP or Hs ClpP protein and various concentrations of compound was added into the system. After an incubation at 37 °C for 2 h, samples were mixed with SDS loading buffer and heated at 100 °C for 10 min. Then the samples were loaded to the SDS-PAGE for detecting cellular Sa FtsZ abundance. The proteins were transferred to nitrocellulose membrane (Millipore) and blocked with TBST containing 5% skim milk at room temperature for 1 h, followed by incubation with the primary antibodies of Sa FtsZ (1:5,000) and Sa GAPDH (1:5,000) at 4 °C overnight. After washing with TBST, HRP-labeled goat anti-rabbit IgG (1:10,000) was added for Western Blot analysis. Differential scanning fluorimetry (DSF) The Sa ClpP or Sa ClpPI91W protein was dissolved in 100 mM HEPES, pH 7.0, 100 mM NaCl to a final concentration of 2 μM (monomeric concentration), while Hs ClpP, Hs ClpPΔC, Hs ClpPW146A or Hs ClpPW146AΔC was dissolved into the assay buffer containing 20 mM Tris-HCl, pH 7.5, 500 mM NaCl, and 5% glycerol to a final concentration of 2 μM (monomeric concentration). Compounds in varying concentrations (containing 1% DMSO) were added into the assay buffer. After incubation at room temperature for 10 min, 5 × SYPRO Orange dye (Invitrogen) was added into each sample. The detection was recorded in a CFX96 Real-Time System (Bio-Rad) at the wavelength of 492 nm for excitation and 610 nm for emission. The samples were heated from 25 °C to 95 °C at a rate of 1 °C/min. Data analysis was performed with Bio-Rad CFX Manager software and GraphPad Prism 8. The T m of proteins in compound-treated groups were referenced against that in DMSO group. Isothermal titration calorimetry (ITC) ITC experiments were performed in a buffer containing 20 mM HEPES, 100 mM NaCl, pH 7.0, 5% DMSO at 25 °C and with constant stirring at 750 rpm on a MicroCal iTC200 system (GE Healthcare) according to the reported method [44] , [60] . The proteins and compounds were dissolved in the exact same buffer. The cell was filled with 50 μM ( R )- or ( S )- ZG197, and the syringe was filled with Sa ClpPI91W at 500 μM or Sa ClpP at 700 μM. After an automatic equilibration of system, 2 μL solution in syringe was injected into the cell to trigger binding reaction and producing the characteristic peak sequence in the recorded signal. Data analysis including baseline correction and evaluation was carried out with OriginPro 8.5 ITC. Fits were carried out considering all injections except the first injection to calculate the maximum heat and the value of equilibrium dissociation constant ( K d ). Biolayer interferometry (BLI) assay This experiment was performed using Octet RED96 (ForteBio). The Sa ClpP and Hs ClpP proteins were biotinylated in PBS buffer at room temperature for 1 h. Then the biotinylated proteins were collected using a PD MiniTrap™ G-25 Desalting Column (cytiva). The streptavidin biosensors were incubated in PBST (PBS with 0.5% Tween-20) containing 0.5% DMSO for 10 min followed by loading with 50 μg/mL biotinylated Sa ClpP or Hs ClpP. The reference control applied a duplicate set of sensors that was incubated only in PBST with 0.5% DMSO. Various concentrations of ( R )- and ( S )-ZG197 were used to calculate the binding curve. The detection was conducted with a standard protocol in 96-well black plates with a total volume of 200 μL at 30 °C. BLI data were collected using Octet Acquisition 11.0. The signals were analyzed by a double reference subtraction protocol to calculate the binding kinetics using Octet Analysis 11.0. The K d values were calculated from the steady-static fit curve. Plasmid construction and protein overexpression in S. aureus To construct the plasmid for the constitutive expression of Sa ClpP in S. aureus , a DNA fragment, covering the clpP gene and its upstream 29 base pairs, was amplified from S. aureus 8325-4 genomic DNA and cloned into pYJ335. The SaclpPI91W mutant was constructed according to QuikChange II site-directed mutagenesis kit with primers Sa clpPI91W-F and Sa clpPI91W-R. For plasmid maintenance, 100 μg/mL ampicillin was used in E. coli , and 10 μg/mL erythromycin was used in S. aureus . The plasmid was extracted from DH5α and subsequently transformed into electrocompetent S. aureus RN4220, from which the plasmid was extracted again and finally transformed into electrocompetent S. aureus 8325-4/Δ clpP cells. Erythromycin was used at 10 µg/mL for plasmid selection, and 1 ng/mL ATC was added to induce protein expression. SaclpP -F1 primer: GTAACAGTTATTACAAGGAGG SaclpP -R1 primer: AGGGGGCCCTTATTTTGTTTCAGG SaclpPI91W -F primer: GATGTTCAAACATGGTGTATCGGTATGGC SaclpPI91W -R primer: GCCATACCGATACACCATGTTTGAACATC The protein overexpression was detected using Western blot. An overnight culture of bacteria was diluted at 1:1000 in TSB with aeration at 220 rpm. When OD 600 reached 0.6, 1 mL culture was collected and centrifuged at 12,396 × g for 3 min. The sediments were washed with PBS for three times and resuspended in 100 μL PBS with 0.75 U Lysostaphin (Sigma) at 37 °C for 30 min. The samples were then centrifuged at 12,396 × g , 4 °C for 30 min and the supernatants were collected. Protein concentration was quantified with BCA Protein Assay Kit (Beyotime). The samples were diluted with SDS loading buffer, heated at 100 °C for 10 min, and loaded to the SDS-PAGE for analysis. The proteins were transferred to nitrocellulose membrane (Millipore) and blocked with TBST containing 5% skim milk at room temperature for 1 h, followed by incubation with the primary antibodies of Sa ClpP (1:5,000) and Sa GAPDH (1:5,000) at 4 °C overnight. HRP-labeled goat anti-rabbit IgG (1:10,000) was then added. The enhanced chemiluminescence (ECL) was used to autoradiography, and the images were captured with GE ImageQuantLAS4000. Sa FtsZ degradation in intact cells S. aureus 8325-4 strains with genetic backgrounds of clpP , Δ clpP , and the complemented clpP or I91W mutant were assayed for Sa FtsZ degradation in intact cells. An overnight culture was diluted at 1:200 and incubated with varying concentrations of each compound (0, 5, 10, and 20 μM, final concentration of DMSO at 1%). When OD 600 reaches 0.7, 300 μg/mL spectinomycin was added and the reaction was conducted at 37 °C, 220 rpm for 3 h. Then 1 mL of each sample was taken and washed with PBS three times. The cells were resuspended and lysed with 0.75 U Lysostaphin at 37 °C for 30 min. The supernatant of lysed cell extracts was separated, and proteins’ concentration were determined using BCA Protein Assay Kit followed by Western blot analysis. Quantitative analysis was performed using ImageJ software. Degree of Sa FtsZ degradation was determined by measuring the band intensity of Sa FtsZ against Sa GAPDH and the DMSO panel was considered as 1.0. Screening for the resistant mutants Single colonies of S. aureus 8325-4 were picked up and grown at TSA with shaking overnight. The culture was diluted with 1:1000 and grown to OD 600 = 0.6. Then the culture was resuspended in PBS and 5 × 10 6 cells were spread on MHA plates containing ( R )-ZG197, ( S )-ZG197, ADEP 4 or ONC212 at 4 × MIC of each compound. After 24 h, resistant colonies were randomly picked for MIC determinations and sequencing. The SaclpP gene was amplified by PCR and sequenced for determining the mutant site. The sequences of the primers used for amplifying SaclpP are shown as follows: SaclpP -F2 primer: GTTATTACAAGGAGGAAAT SaclpP -R2 primer: CAGACAGCTTAGTCTACTC Scanning electron microscopy (SEM) Overnight cultures of S. aureus strains were diluted at 1:200 in fresh TSB medium and incubated with DMSO or 20 μM ( R )- and ( S )-ZG197 then shaken at 37 °C, 220 rpm for 3 h. The cultures were washed by PBS three times and resuspended to OD 600 of 1.5. Then 50 μL of cultures were taken and fixed on 13 mm cover glass with 300 μL 2.5% glutaraldehyde (TED PELLA) in 24 well plate (Corning) at 4 °C overnight. On the next day, the glutaraldehyde in each well was removed and washed with PBS three times. Then the samples were dyed with osmic acid carefully for 30 min followed by washing with ddH 2 O three times. Samples were dehydrated in a graded series of ethanol (30, 50, 70, 80, 95, 100%) for 10 min with gentle shaking for each step. Samples were then subjected to critical point drying with liquid CO 2 (Leica EM) to maintain original appearance of samples. Dried samples were coated with a gold film by sputter coating (Leica EM). Samples were imaged in a FEI Quanta 250 at an acceleration voltage of 15 kV. Images were recorded and contrast and brightness were adjusted with Adobe Photoshop CS5. Cellular thermal shift assay (CETSA) Overnight cultures of S. aureus 8325-4 or the rescued SaclpPI91W strains were diluted at 1:200 in fresh TSB and were incubated with DMSO or 10 μM compounds, including ( R )-ZG197, ( S )-ZG197, and ONC212, for 2 h. One milliliter of each culture was collected and washed with PBS for three times. Then the samples were resuspended in PBS containing cocktail inhibitors (Sangon Biotech) and divided into 50 μL aliquots and heated at different temperatures for 3 min using a thermal cycler (BIO-RAD). The bacteria were then lysed with 0.75 U Lysostaphin at 37 °C for 30 min followed by three freeze-thaw cycles with liquid nitrogen to crack bacteria completely. The soluble lysates were collected by centrifugation at 12,396 × g for 20 min at 4 °C and the supernatants were analyzed by Western blot. Primary antibodies of Sa ClpP (1:5,000) and Sa GAPDH (1:5,000) were used. Three independent experiments were performed, and one of the representative results is shown. HEK 293 T/17 cells were digested by trypsin and collected. The cell sediments were resuspended in PBS containing cocktail inhibitors (Sangon Biotech) and lysed by three freeze-thaw cycles with liquid nitrogen. The lysed samples were then centrifuged at 12,396 × g for 30 min to remove the debris. After centrifugation, the supernatant was incubated with 10 μM compounds, including ( R )-ZG197, ( S )-ZG197, and ONC212, for 20 min and then transferred into the 0.2 mL PCR tubes followed by denaturing at indicated temperatures for 3 min. Then the soluble supernatants were collected by centrifugation and were analyzed by Western blot. Primary antibodies of Hs ClpP (1:2,000) and β-actin (1:5,000) were used. Three independent experiments were performed, and one of the representative results is shown. Minimum inhibitory concentration (MIC) assay Cultures were grown in MHB medium at 37 °C with shaking at 220 rpm from overnight until OD 600 reached 0.4-0.6, and then diluted into MHB medium to give a final OD 600 of 0.025. Compounds at various concentrations were added to diluted bacterial cultures (100 µL/well final volume and final DMSO concentration of 1%) in triplicates. The lowest concentration of an antibiotic that inhibited the visible growth of bacteria was recorded after incubation at 37 °C for 18 h. MIC values were determined by three independent experiments. Time killing assay An overnight culture of USA300 was diluted in TSB with a final OD 600 of 0.025 and cultivated to mid-logarithmic phase (OD 600 of 0.6) at 37 °C, 220 rpm. Subsequently, cells were diluted to 1 × 10 6 CFU/mL in TSB and treated with DMSO, vancomycin (20 μg/mL, 10 × MIC), ( R )-ZG197 (5 μg/mL, 10 × MIC), ( S )-ZG197 (80 μg/mL, 10 × MIC), or ONC212 (5 μg/mL, 10 × MIC). After 6 h incubation at 37 °C, 220 rpm, 200 μL culture medium was taken and washed with PBS for three times. Dilutions of each condition were then plated in the absence of compounds and grown on TSA plates at 37 °C overnight. CFUs were measured by counting the number of colonies on the next day. MRSA persister cell assay Two assays were performed to test effects of ( R )- and ( S )-ZG197 on eradicating MRSA persisters. First, S. aureus cells growing at stationary phase were applied [61] . After overnight culturing, stationary phase MRSA USA300 were prepared in BHI broth and incubated in the presence of ( R )-ZG197 (10 μg/mL), ( S )-ZG197 (80 μg/mL), ciprofloxacin (8 μg/mL), or rifampicin (0.4 μg/mL) at 37 °C and 220 rpm with aeration. At each indicated time point (0, 24, 48, and 72 h), 100 μL of culture was taken and centrifuged at 12,396 × g for 2 min. Then the mixture was washed with PBS for three times. 10-fold serial dilutions were performed and 10 μL of each dilution was removed and spotted onto TSA plates. All plates were placed at 37 °C overnight. CFUs were measured by counting the number of colonies on the next day. The second persister cell assay was performed using the biphasic killing analysis [23] . Overnight, stationary-phased USA300 culture was diluted at 1:100 in TSB. Bacteria were first incubated with ciprofloxacin (8 μg/mL, 10 × MIC) for 6 h at 37 °C with aeration at 220 rpm, and the remaining cells formed surviving persisters. Then compounds at 10 × MIC, including ( R )-ZG197 (10 μg/mL), ( S )-ZG197 (80 μg/mL), ADEP 4 (5 μg/mL), ciprofloxacin (8 μg/mL), or rifampicin (0.4 μg/mL), were added and 100 μL samples were taken at indicated time point (0, 2, 4, 6, 8, 12, 24, and 48 h) and centrifuged at 12,396 × g for 2 min. Then samples were resuspended in PBS. CFUs were measured by counting the number of colonies on the next day. Cytotoxicity assay The toxicity of the compounds on 293T/17 and HK-2 cell lines was performed by 3-(4,5-dimethylthiazol-2-yl)-2,5-diphenyltetrazolium bromide (MTT) assay. Mammalian cells (3000 cells/well) were seeded in 96-well plates allowed to adhere overnight and treated with a diluted series of ICG-001, ( S )-ZG197, ( R )-ZG197, or ONC212 for 72 h. Subsequently, 10 μL prepared MTT solution (5 mg/mL in PBS) was added to each well and the cells were then incubated for another 4 h at 37 °C. After removing the supernatant, the formazan precipitate in each well was dissolved in DMSO and the absorbance was measured at a wavelength of 490 nm by Tecan Spark 10 m plate reader. DMSO was used as a control and its viability was considered as 100%. IC 50 values were calculated by fitting dose−response curves. All experiments were performed in triplicate. Wnt/β-catenin luciferase reporter assay Wnt/β-catenin signaling was detected using TOPFlash/FOPFlash reporter assays as previously described with modifications [39] . TOPFlash (#21-170, Millipore) was used as a Wnt-responsive reporter and FOPFlash (#21-169, Millipore) was a mutant Wnt-irresponsive reporter. About 1.5 × 10 5 HEK 293 T/17 or HK-2 cells were seeded in 24-well plates. After attachment, cells were transfected with 500 ng Firefly reporter TOPFlash or FOPFlash using Lipofectamine 2000 (Invitrogen, USA) according to manufacturer’s instructions. Meanwhile, 50 ng of the Renilla reporter pRL-TK (Promega) was co-transfected as an internal control to correct for differences in both transfection and harvest efficiencies. After 6 h post-transfection, the culture medium was changed into DMEM growth medium in the presence of 20 mM LiCl and compounds at indicated concentrations. After 24 h, cells were lysed and detected by Dual-Luciferase Reporter Assay System (#E1910, Promega) according to manufacturer’s instructions. The Firefly luciferase activity (TOPFlash or FOPFlash) were normalized with Renilla luciferase activity (pRL-TK). Wnt signaling activity was represented as normalized TOPFlash/FOPFlash values. Zebrafish infection model Zebrafish (7 to 11 months old, 300 ± 50 mg, regardless of gender) were maintained in a 10-L tank with regular feeding for at least three days before subjecting to experiments. The safety profiles were conducted by intraperitoneally injecting the uninfected zebrafish ( n = 11 per group) with 25, 50, or 100 mg/kg compounds (dissolved in 5% DMSO, 20% PEG 300, 5% solutol, and 70% PBS). For determination of an appropriate staphylococcal load for infection, zebrafish were administered with a serial CFUs of bacteria and the survival rates were monitored over 5 days. One group zebrafish was intraperitoneally injected with the same volume of PBS (8 μL) as blank control. For investigation on anti-infective efficacy of compounds, the zebrafish were intraperitoneally injected with S. aureus strains (USA300, Newman, Newman Δ clpP or MRSA XJ049) at indicated CFUs. After 30 min post infection, zebrafish were divided randomly into different groups followed by administration of compounds at a dose of 25 or 50 mg/kg and vehicle control. Survival rates of zebrafish were recorded for 5 days. Murine skin infection model The infection model was established according to previously reported method with some modifications [62] . The backs of mice (6 to 8 weeks old, 18-20 g) were shaved and treated with depilatory cream one day before infection. Overnight cultures of S. aureus USA300 were diluted at 1:1000 and grown to OD 600 at 0.6. Then cultures were washed by PBS three times and resuspended at a concentration of 5 × 10 7 CFU/mL. Before infection, mice were anesthetized with an intraperitoneal injection of 70 mg/kg pentobarbital sodium. An aliquot of 50 µL S. aureus USA300 suspension (containing 2.5 × 10 6 CFUs) were subcutaneously injected into the shaved area. At 16 h post infection, mice were randomly divided into different groups ( n = 9 per group). The lesion area was measured and calculated using the formula A = π( L /2) × W /2 ( A , area; L , length; W , width). The difference of the initial lesion areas has no significance in each group. Then 50 µL of 7.5 mg/kg compounds (dissolved in 5% DMSO, 20% PEG 300, 5% solutol, and 70% PBS) and vehicle (as negative control) were subcutaneously injected near the infected skin. The treatments were applied twice daily for 3 days. Mice were then sacrificed and the skin was separated from the underlying fascia and muscle tissue. One of the nine skin samples in each group was randomly used and fixed in 4% paraformaldehyde and embedded in paraffin. Thin sections were cut and stained with H&E for microscopic observations. The remaining eight infected skin samples in each group were aseptically excised and weighed, and subsequently homogenized in 1 mL of PBS. The serially diluted homogenate was plated onto TSA plates and incubated at 37 °C overnight. 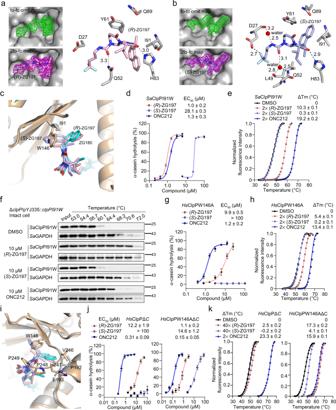Fig. 4: Identification of key sites/motif for selectiveSaClpP overHsClpP activation. Close view of interactions of (R)- (a) and (S)-ZG197 (b) in the hydrophobic site ofSaClpP. The fo-fc omit map for showing (R)- and (S)-ZG197 binding is contoured at 3.0 Å and colored in green, while the 2fo-fc map is contoured at 1.0 Å and colored in magenta, respectively. (R)- and (S)-ZG197 are colored in light pink and light blue, respectively. Hydrogen bonds are indicated by dark dashed lines, and the distance is labeled in Å.cClose view of structural alignments of (R)- and (S)-ZG197 bound toSaClpP complexes, and ZG180 bound toHsClpP in the hydrophobic pockets. ZG180, (R)- and (S)-ZG197 are colored in cyan, light pink, and light blue, respectively.SaClpP is colored in gray, whileHsClpP is colored in wheat.dQuantitation of α-casein hydrolysis by theSaClpPI91W mutant in the presence of (R)-ZG197, (S)-ZG197, and ONC212, respectively.eEffect of activators on the thermal stability of theSaClpPI91W protein detected in the DSF assay.fRepresentative Western blot images showing the effects of 10 μM activators on the thermal denaturation of theSaClpPI91W protein in intact cells of the complementedclpPI91Wmutant strain.SaClpPI91W expression was induced in the presence of anhydrous tetracycline (ATC) at 1 ng/mL. Three biological replicates were performed for each experiment.gQuantitation of ClpP activators-promoted hydrolysis of α-casein by theHsClpPW146A mutant.hEffect of activators on the thermal stability of theHsClpPW146A mutant detected in the DSF assay.iClose view of the structural alignment in (c) shows the effect of the C-terminal residues on activators’ binding and activation ofHsClpP.jQuantitation of effect of activators-activated α-casein hydrolysis by theHsClpPΔC (left) andHsClpPW146AΔC (right) truncations, respectively.kEffect of activators on the thermal stability of theHsClpPΔC (left) andHsClpPW146AΔC (right) detected in the DSF assay Data (d,e,g,h,j, andk) are obtained from three biologically independent experiments and presented as mean ± SD (error bars). Source data are provided as a Source Data file. The bacterial counts were expressed as log 10 CFUs/mg of tissue. Statistics and reproducibility All statistical analyses were performed using GraphPad Prism 8 (GraphPad software). Log-rank tests were performed to compare the two survival curves. Two-tailed unpaired Student’s t-tests were performed to compare the means between groups. Data are presented as mean ± SD. P values are indicated in the figures. The number of independent experiments/mice/samples are mentioned in the figure legends. All attempts at replication are successful. All blots and gels were performed in triplicate and a single experimental image is shown. Murine skin infection experiments, SEM and H&E staining were performed once. At least 5 representative images of SEM were recorded from each sample. 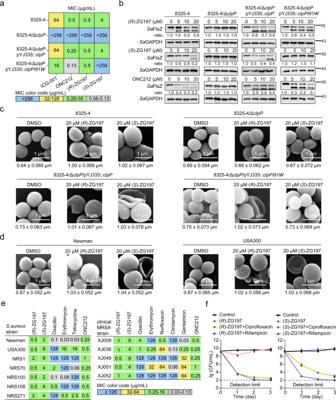Fig. 5: Target dependency of (R)- and (S)-ZG197’ antibacterial activity in cellular contexts. aAssessment of ClpP activators on the growth ofS. aureus8325-4 with genetic backgrounds ofclpP, ΔclpP, and complementedclpPorI91Wmutant by MIC measurement.bAssessment ofSaClpP activators’ effect on the cellularSaFtsZ abundance in the intact cells of 8325-4, ΔclpP, the complementedclpPandclpPI91Wstrains detected in Western blot. Quantitation on the band intensity ofSaFtsZ is normalized against the loading control ofSaGAPDH, and the ratio in the DMSO group is considered as 1.0.cRepresentative views of SEM micrographs showing the effects of (R)- and (S)-ZG197 on the cell morphology ofS. aureus8325-4 having different genetic backgrounds ofclpP, ΔclpP, and complementedclpPorclpPI91W. The scale bar represents 1 μm.dRepresentative views of SEM micrographs showing the effect of 20 µM (R)- and (S)-ZG197 on cell division of Newman and USA300 strains. The scale bar represents 1 μm.eDetermination of MIC of theSaClpP activators against the growth of a panel ofS. aureusstrains. (R)- and (S)-ZG197, ONC212, and the clinic antibiotics oxacillin, tetracycline, erythromycin, norfloxacin, clindamycin, and gentamicin were assayed under similar conditions. The experiments were performed in triplicates.fBactericidal effect of (R)- and (S)-ZG197 combined therapy on eradicating stationary phase USA300 (n= 3 biologically independent experiments). Cell numbers were recorded in CFU/mL. Data are presented as mean ± SD. Source data are provided as a Source Data file. 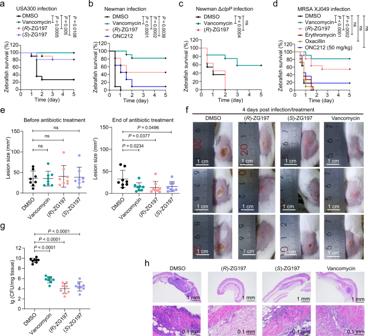Fig. 6: Anti-infective effects of (R)- and (S)-ZG197 in vivo. aTherapeutic effect of (R)- and (S)-ZG197 against USA300 infection in zebrafish. Zebrafish (n= 11 animals) were infected with 7 × 106CFU of USA300, and compounds were administered at a single dose of 50 mg/kg. DMSO (5%) and vancomycin were administered as controls. Therapeutic effect of (R)-ZG197 against lethal infection by Newman (b) and the ΔclpPmutant (c). Zebrafish (n= 11 animals) were infected with 7 × 107CFU of Newman (b) or 3 × 107CFU of the ΔclpPmutant (c), and compounds were administered to infected zebrafish at 50 mg/kg. Vancomycin and ONC212 were used as controls.dTherapeutic effect of (R)-ZG197 on the clinical MRSA isolates infected zebrafish. Zebrafish (n= 11 animals) were infected with 5 × 107CFU of XJ049, and compounds were administered at a single dose of 50 mg/kg. DMSO (5%), antibiotics (vancomycin, erythromycin, and oxacillin), and the global activator ONC212 were used as controls.eQuantitation of necrotic skin lesion size of initial (left panel) and 4 days post-infection (right panel). Vancomycin was used as a positive control. Data are shown as mean ± SD (n= 9 animals).fRepresentative images showing necrotic skin lesions 4 days post-infection. The scale bar represents 1 cm.gEffects of our activators on bacterial counts in the skin samples (n= 8 biologically independent samples). Skin tissue was excised from mice infected with USA300 4 days post-infection and plated onto TSA to enumerate CFUs.hMicrographs of H&E-stained skin tissues after the indicated treatments. The scale bar represents 1 mm (Top) and 0.1 mm (Bottom). Statistical differences were analyzed using Log-rank tests (a–d) and two-tailed unpaired Student’st-tests (e,g). ExactPvalues are provided. ns, no significance. Data (e,g) are presented as mean ± SD (error bars). Source data are provided as a Source Data file. Three representative images of H&E staining were taken in each sample and one is shown. All images recorded on SEM or H&E staining indicated a similar trend. Reporting summary Further information on research design is available in the Nature Portfolio Reporting Summary linked to this article.